Nanoporous gold supported cobalt oxide microelectrodes as high-performance electrochemical biosensors Tremendous demands for electrochemical biosensors with high sensitivity and reliability, fast response and excellent selectivity have stimulated intensive research on developing versatile materials with ultrahigh electrocatalytic activity. Here we report flexible and self-supported microelectrodes with a seamless solid/nanoporous gold/cobalt oxide hybrid structure for electrochemical nonenzymatic glucose biosensors. As a result of synergistic electrocatalytic activity of the gold skeleton and cobalt oxide nanoparticles towards glucose oxidation, amperometric glucose biosensors based on the hybrid microelectrodes exhibit multi-linear detection ranges with ultrahigh sensitivities at a low potential of 0.26 V (versus Ag/AgCl). The sensitivity up to 12.5 mA mM −1 cm −2 with a short response time of less than 1 s gives rise to ultralow detection limit of 5 nM. The outstanding performance originates from a novel nanoarchitecture in which the cobalt oxide nanoparticles are incorporated into pore channels of the seamless solid/nanoporous Au microwires, providing excellent electronic/ionic conductivity and mass transport for the enhanced electrocatalysis. Electrochemical biosensors, which have been widely employed in clinical, environmental, industrial and agricultural applications, recognize biological analytes through a catalytic or binding event occurring at the interface of electrodes [1] , [2] , [3] , [4] , [5] . Intimate correlation of biosensing performance and the electrocatalytic and structural properties of electrodes has stimulated considerable efforts devoted to innovational materials to coordinate mass- and charge-transport and electron-transfer kinetics for realizing simultaneous minimization of primary resistances in biosensing: electrochemical reaction occurring at electrolyte/electrode interface, mass transport of analyte in electrolyte and electrode, and the electron conduction in electrode and current collector [6] , [7] , [8] , [9] . Nanostructured metal oxides have promising applications as nonenzymatic catalysts in new generation of miniaturized glucose biosensors owing to their low cost, high biocompatibility and electrocatalytic activity, as well as enhanced electron-transfer and adsorption capacities [10] , [11] . Judicious use of nanostructured metal oxides is expected to circumvent the key limitations of expensive enzymes, typically glucose oxidase (GOx), with compromise of the sensitivity, reproducibility and stability of glucose detection as the catalytic activity of GOx is intrinsically susceptible to environmental conditions such as temperature, humidity, pH and toxic chemicals [2] , [11] , [12] , [13] . However, the poor electronic conductivity of metal oxides (for example, Co 3 O 4 in ~10 −5 S m −1 at room temperature) significantly impedes them from wide use in electrochemical biosensing devices with high sensitivity and reliability, fast response and excellent selectivity [10] , [14] , [15] . One of major strategies to enhance charge transport in electrochemical biosensors is to design composite materials by combining highly electrocatalytic materials with a conductive substance [16] , [17] , [18] , [19] , [20] , whereas single- and multi-walled carbon nanotubes (CNTs) [21] , [22] , [23] , [24] , [25] , graphene [26] , [27] and noble metal nanoparticles [28] have been explored to serve as conductive pathways of metal oxides (TiO 2 , MnO 2 , RuO 2 , Co 3 O 4 and NiO). Although these low-dimensional composite nanostructures could provide extremely large specific surface area of the electrode/electrolyte interface [16] , [17] , [18] , [19] , [20] , [21] , [22] , [23] , [24] , [25] , [26] , [27] , [28] , the assembled electrodes exhibit an undesirably low electronic conductance as a consequence of exceptionally low electron transport in the nanomaterials as well as the high contact resistances within nanomaterials and between the current collector and electrodes [29] , [30] , greatly hindering their potential applications in electrochemical biosensors at ultralow concentrations in unconventional body fluids. Here we report multifunctional seamless solid/nanoporous Au/Co 3 O 4 (S/NPG/Co 3 O 4 ) hybrid microelectrodes with three-dimensional (3D) bicontinuous nanoporosity, facilely fabricated by incorporating Co 3 O 4 nanoparticles onto seamless solid/nanoporous Au (S/NPG) microwires, for nonenzymatic electrochemical glucose biosensors. Amperometric measurements at a low potential demonstrate that the seamless S/NPG/Co 3 O 4 microelectrodes can detect ultralow-concentration glucose with an ultrahigh sensitivity of ~12.5 mA mM −1 cm −2 and a fast response time of <1 s. The outstanding sensing performance results from the unique nanoarchitecture, which simultaneously minimizes the contact resistances among current collector of solid Au wire, nanoporous Au skeleton and Co 3 O 4 nanoparticles. Furthermore, the nanoarchitecture provides interconnected nanoporous channels and Au ligaments, concurrently enhancing the transports of glucose and electron, and offers a large specific surface area of electrode/electrolyte interface, facilitating the full use of the enhanced electrocatalysis of Au/Co 3 O 4 hybrid. Synthesis and characterization Our fabrication strategy briefly illustrated in Fig. 1 is to combine the alloying/dealloying and hydrothermal methods, through which the preparation of seamless S/NPG microwires and the incorporation of Co 3 O 4 nanoparticles into the nanopore channels are consecutively carried out. The Au microwires of 200-μm-diameter with seamless solid/nanoporous architecture ( Fig. 2a ) are produced by in situ electrochemical alloying/dealloying protocol in an electrolyte composed of ZnCl 2 and benzyl alcohol (BA) [31] , during which Au–Zn alloys are firstly formed via the electrodeposition of zinc, and the less noble Zn is then selectively dissolved in the dealloying process for the formation of nanoporous layer with high surface area ( Supplementary Fig. S1 ) [32] . The alloying/dealloying conditions ( Supplementary Table S1 ) are adjusted to manipulate the resulting microstructure of nanoporous layer ( Fig. 2 and Supplementary Figs S2–S5 ). Figure 2b shows representative cross-sectional and top-view scanning electron microscope images of the seamless S/NPG microwire, respectively, that is fabricated at the optimized alloying/dealloying conditions in a mixture of BA and 1.5 M ZnCl 2 at a scan rate of 10 mV s −1 and 120 °C (the first conditions in Supplementary Table S1 ). 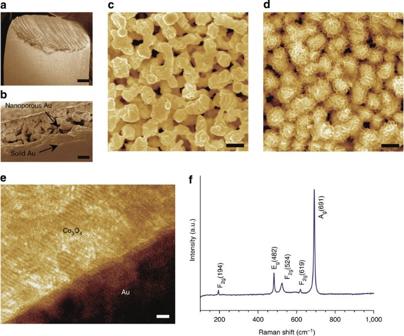Figure 2: Microstructure characterization. (a) Low-magnification and (b) cross-section SEM images of seamless S/NPG microwire. (a) Scale bar, 25 μm; (b) scale bar, 300 nm. Top-view SEM images of (c) bare S/NPG and (d) S/NPG/Co3O4hybrid with the characteristic length of ~300 nm. (c,d) Scale bar, 300 nm. (e) High-resolution transmission electron microscope (HRTEM) image of Au/Co3O4interfacial structure. (e) Scale bar, 2 nm. (f) Surface-enhanced Raman spectrum of seamless S/NPG/Co3O4hybrid microwire. The seamless solid/nanoporous structure possesses ~1 μm thick nanoporous layer ( Fig. 2b ), where a uniform and 3D bicontinuous nanoporous structure consists of quasi-periodic nanopore channels and Au ligaments with characteristic length of ~300 nm ( Fig. 2c and Supplementary Fig. S6 ) [32] , [33] . 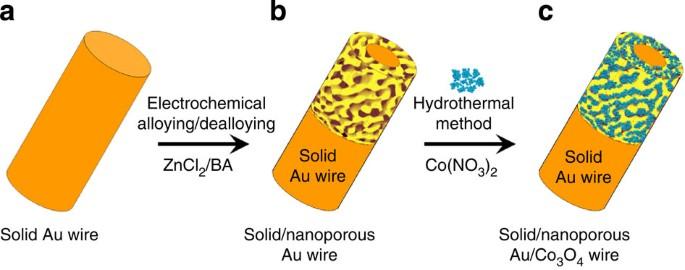The decreases of the cycle number, temperature, ZnCl 2 concentration and scan rate in the alloying/dealloying process ( Supplementary Table S1 ) will reduce the thickness and characteristic length of nanoporous layer and change the real surface area of S/NPG skeleton, as demonstrated by scanning electron microscope micrographs and in situ electrochemical measurements ( Supplementary Figs S2–S5,S7a and Supplementary Notes 1,2 ) [34] . Figure 1: Scheme for fabrication of hybrid microelectrodes. (a) Solid gold microwire. (b) 3D bicontinuous nanoporous gold layer is formed directly on the solid gold microwire by electrochemical alloying/dealloying in a mixed electrolyte of BA and ZnCl2. (c) Co3O4nanoparticles are decorated onto nanopore channels of seamless S/NPG microwire by a hydrothermal method in a mixed solution containing Co(NO3)2. Figure 1: Scheme for fabrication of hybrid microelectrodes. ( a ) Solid gold microwire. ( b ) 3D bicontinuous nanoporous gold layer is formed directly on the solid gold microwire by electrochemical alloying/dealloying in a mixed electrolyte of BA and ZnCl 2 . ( c ) Co 3 O 4 nanoparticles are decorated onto nanopore channels of seamless S/NPG microwire by a hydrothermal method in a mixed solution containing Co(NO 3 ) 2 . Full size image Figure 2: Microstructure characterization. ( a ) Low-magnification and ( b ) cross-section SEM images of seamless S/NPG microwire. ( a ) Scale bar, 25 μm; ( b ) scale bar, 300 nm. Top-view SEM images of ( c ) bare S/NPG and ( d ) S/NPG/Co 3 O 4 hybrid with the characteristic length of ~300 nm. ( c , d ) Scale bar, 300 nm. ( e ) High-resolution transmission electron microscope (HRTEM) image of Au/Co 3 O 4 interfacial structure. ( e ) Scale bar, 2 nm. ( f ) Surface-enhanced Raman spectrum of seamless S/NPG/Co 3 O 4 hybrid microwire. Full size image Seamless S/NPG/Co 3 O 4 hybrid microwires are synthesized by the hydrothermal method ( Supplementary Table S1 ), wherein the loading amount and morphology of Co 3 O 4 can be tailored by the Co(NO 3 ) 2 concentration ( Supplementary Fig. S8 ) and the heating temperature ( Supplementary Fig. S9 ), respectively. At a constant hydrothermal temperature of 180 °C, the loading amount of Co 3 O 4 increases with the increasing concentration of Co(NO 3 ) 2 ( Supplementary Fig. S8 ). In the mixed solution containing 6 mM Co(NO 3 ) 2 , the well-crystallized Co 3 O 4 nanoparticles uniformly and directly grow into nanopores along the Au ligaments of the seamless S/NPG microwires ( Fig. 2d and Supplementary Fig. S10 ). The rough Co 3 O 4 nanoparticles are composed of nanocrystals with diameter of ~5–20 nm, giving rise to a larger real surface area of S/NPG/Co 3 O 4 than that of bare S/NPG ( Fig. 2e and Supplementary Fig. S7 ). When the hydrothermal temperature increases to 260 °C, nanosheet-shaped Co 3 O 4 grows vertically on Au ligaments ( Supplementary Fig. S9a ), whereas at 100 °C, the formation of Co 3 O 4 film seals the nanoporous structure of hybrid microelectrode ( Supplementary Fig. S9c ), significantly reducing the available electrolyte/electrode interface ( Supplementary Fig. S7b and Supplementary Note 1 ). The high-resolution transmission electron microscope image of Au/Co 3 O 4 interface ( Fig. 2e ) indicates that the Co 3 O 4 nanoparticles have end-bonded contacts with the Au ligaments [29] , offering excellent electrical conductivity between Au and Co 3 O 4 . The characteristic peaks at 194, 482, 524, 619 and 691 cm −1 in the surface-enhanced Raman spectrum of Co 3 O 4 , which are assigned to the F 2g , E g , F 2g , F 2g and A 1g vibrational modes, respectively, unveils a spinel-type crystalline structure ( Fig. 2f ) [35] , [36] . This is further confirmed by the obvious diffraction peaks in X-ray diffraction pattern of S/NPG/Co 3 O 4 hybrid corresponding to the (220), (311), (222), (400), (422), (511) and (440) planes of spinel-type Co 3 O 4 (JCPDS 42–1467) [27] , apart from two significant diffraction peaks at 2 θ =44.4° and 77.6° attributed to the (200) and (311) reflections of Au (JCPDS 65–2870) ( Supplementary Fig. S11 ). The direct decoration of 3D bicontinuous nanoporous Au layer on the Au microwires facilitates the integration of nanoporous metal/oxide composites with current collectors without any additional contact resistance [37] . By this technology, the entire assembled electrode not only retains excellent electrical conductivity up to the Au bulk value (~4 × 10 5 S cm −1 ), much higher than those of conventional electrodes based on conducting polymers and various carbon materials, but exhibits exceptional mechanical flexibility ( Supplementary Fig. S12 ). Electrocatalytic activity for glucose oxidization To assess their electrocatalytic activity, self-supported seamless S/NPG and S/NPG/Co 3 O 4 microwires as well as Co 3 O 4 nanoparticles (size ~5–20 nm, similar to those grown on seamless S/NPG microwire) on an ITO glass substrate ( Supplementary Fig. S13a ) are directly used as working electrodes for cyclic voltammetry measurements. In a N 2 -bubbled mixture of 0.5 M KOH and 10 mM glucose at a scan rate of 20 mV s −1 , the cyclic voltammograms (CVs) for the S/NPG/Co 3 O 4 microelectrodes synthesized under various alloying/dealloying and hydrothermal conditions ( Supplementary Table S1 ) are acquired, as shown in Fig. 3 and Supplementary Figs S2d,S3–S5c,S8–S9d . 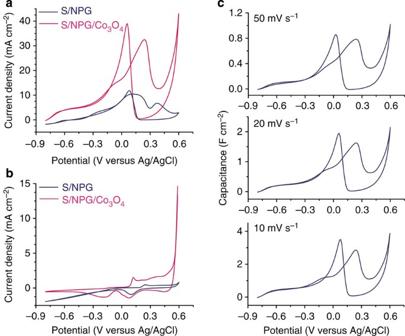Figure 3: Electrochemical characterization. Cyclic voltammetry (CV) curves of seamless S/NPG and S/NPG/Co3O4hybrid microelectrodes in 0.5 M KOH (a) with and (b) without 10 mM glucose at a scan rate of 20 mV s−1. (c) CV profiles of the seamless S/NPG/Co3O4wire electrode at different scan rates. Current axis incis scaled by the scan rate. Figure 3a illustrates the typical CV for S/NPG/Co 3 O 4 hybrid microelectrode fabricated under the optimized alloying/dealloying and hydrothermal conditions (the first ones in Supplementary Table S1 ), in distinct contrast with its blank voltammetry (without glucose) ( Fig. 3b ) due to the glucose oxidation. In the glucose-free alkaline solution, S/NPG/Co 3 O 4 concurrently presents characteristic features of both Au and Co 3 O 4 nanoparticles. These include the current-density peaks of the oxidation of Au and the more negative subsequent reduction of Au oxides than that of the bare S/NPG microwire ( Fig. 3b ) [38] . In addition, two redox pairs of Co 3 O 4 involve the reversible transition between Co 3 O 4 and CoOOH via Co 3 O 4 +OH − +H 2 O↔3CoOOH+e − and the further conversion between CoOOH and CoO 2 via CoOOH+OH − ↔CoO 2 +H 2 O+e − ( Supplementary Fig. S13b ) [15] , [27] . For comparison, the CVs of the corresponding S/NPG microwire and Co 3 O 4 nanoparticles in 0.5 M KOH with and without 10 mM glucose are also included in Fig. 3a , and Supplementary Fig. S13b , respectively, presenting low electrocatalytic activities [15] , [27] , [38] , [39] . Remarkably, the CV of the seamless S/NPG/Co 3 O 4 hybrid microelectrode shows a much more negative onset potential and higher anodic current density than those of the bare seamless S/NPG microwire and the Co 3 O 4 nanoparticles ( Fig. 3a and Supplementary Fig. S13b ), suggesting synergistic electrocatalytic activity of S/NPG and Co 3 O 4 in the hybrid towards glucose electrooxidation. As shown in Fig. 3a , the voltammetric behaviour of the seamless S/NPG/Co 3 O 4 hybrid microelectrode in the low potential range (<~−0.06 V) produces a substantially enhanced current response as a result of glucose electrosorption [28] , [38] , [40] . This takes place on the significantly increased electroactive surface sites to form the adsorbed intermediates by releasing one proton per glucose molecule at an onset potential of ~−0.78 V (much more negative than ~−0.49 V for bare S/NPG microwire). Accompanying by electrosorption of glucose, the accumulation of the concomitant intermediates on the electrode surface inhabits direct oxidation of glucose on the active sites of Au hence gives rise to the small anodic current peak at ~−0.06 V (refs 28 , 38 , 40 ). Meanwhile, Co 3 O 4 nanoparticles hybridized with seamless S/NPG microwire intervene in a catalytical promotion of glucose oxidation ( Supplementary Fig. S13b ), leading to the continuous increase of the current. At higher positive potentials, both AuOH and CoOOH form on the internal surface of seamless S/NPG/Co 3 O 4 electrode by the partial discharge of OH − , and consequently catalyse the oxidation of intermediates and the direct oxidation of glucose [27] , [28] , [38] , [40] by the conversions of AuOH→Au and CoOOH→Co 3 O 4 , respectively. The corresponding broad anodic current peak is at ~0.25 V. When the potential sweeps more positively, the current density decreases in the potential range of 0.25–0.39 V as formation of Au oxides suppresses the direct electrooxidation of glucose [28] , [38] , [40] . Upon the potential higher than ~0.39 V, the current density dramatically increases as a result of the formation of CoO 2 on which direct glucose oxidation occurs via CoO 2 +C 6 H 12 O 6 →CoOOH+C 6 H 10 O 6 (refs 15 , 27 ). In the negative scan, Au oxides are reduced and a large number of active sites on the internal surface of seamless S/NPG/Co 3 O 4 electrode are regenerated for the direct glucose oxidation, leading to an anodic current peak at ~0.05 V (refs 28 , 38 ). When Co 3 O 4 nanoparticles are incorporated into the S/NPG skeleton with a larger characteristic-length and thinner NPG layer ( Supplementary Note 2 ) at the same hydrothermal conditions ( Supplementary Figs S2–S5 and Supplementary Table S1 ), the CV of S/NPG/Co 3 O 4 hybrid microelectrode shows a lower anodic current density and a less negative onset potential ( Supplementary Figs S2d,S3c–S5c ) because of less surface area for the formation of highly active Au/Co 3 O 4 hybrid ( Supplementary Fig. S7a ). This demonstrates the important role of high nanoporosity of S/NPG skeleton in producing a large amount of Au/Co 3 O 4 hybrid which significantly enhances the electrocatalytic activity of the whole hybrid microelectrodes. Figure 3: Electrochemical characterization. Cyclic voltammetry (CV) curves of seamless S/NPG and S/NPG/Co 3 O 4 hybrid microelectrodes in 0.5 M KOH ( a ) with and ( b ) without 10 mM glucose at a scan rate of 20 mV s −1 . ( c ) CV profiles of the seamless S/NPG/Co 3 O 4 wire electrode at different scan rates. Current axis in c is scaled by the scan rate. Full size image Furthermore, the enhanced electrocatalytic behaviour of seamless S/NPG/Co 3 O 4 hybrid microelectrodes is found to rely significantly on the scan rate ( Fig. 3c ). For lower scan rates, comparatively more glucose is electrooxidized at the surface, indicating a surface-controlled electrochemical process. This is further verified by the observation that the smaller the surface area of S/NPG/Co 3 O 4 microelectrodes, the lower the current densities ( Supplementary Figs S7b,S9d ). It is noteworthy that the change of the surface area results from the evolution of morphology and loading amount of Co 3 O 4 on the same S/NPG microwires at different hydrothermal conditions ( Supplementary Table S1 ). The current density of S/NPG/Co 3 O 4 hydrothermally synthesized at 100 °C falls dramatically as the nanoporous structure is sealed by the Co 3 O 4 film ( Supplementary Fig. S9c,d ), which restrains ion and glucose transports as well as the availability of electrolyte/electrode interface for glucose electrooxidation. Amperometric glucose detection For all S/NPG and S/NPG/Co 3 O 4 microelectrodes ( Supplementary Table S1 ), the glucose sensing performance is evaluated by amperometric measurements, and their current-time curves for successive addition of glucose with concentrations ranging from 1 μM to 10 mM are recorded at an applied potential of 0.26 V ( Fig. 4 and Supplementary Fig. S14 ). As a result of the enhanced electrocatalytic activities of hybrid nanoarchitecture towards glucose oxidation, the current responses and sensitivities of S/NPG/Co 3 O 4 microelectrodes are enhanced by increasing the surface areas of both the S/NPG skeletons and their Co 3 O 4 hybrids ( Supplementary Figs S14,S15 ). The former affords more Au/Co 3 O 4 interface for enhancing the electrochemical activity of Co 3 O 4 and improving the electron transport of Co 3 O 4 to Au network, whereas the latter enables to trap more molecules for electrooxidation and to provide the large surface area of electrolyte/electrode interface for the full use of highly active Au/Co 3 O 4 hybrid. 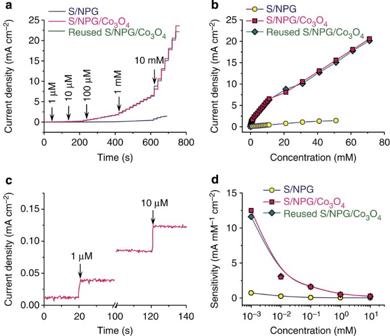Figure 4: Amperometric glucose detection. (a) Chronoamperometry curves and (b) the calibration curves (current density versus glucose concentration) for the amperometric responses of seamless S/NPG and fresh and reused S/NPG/Co3O4microelectrodes to the successive addition of glucose with the concentrations from 1 μM to 10 mM in 0.5 M KOH solution at a constant potential of 0.26 V (versus Ag/AgCl). (c) Fast response of seamless S/NPG/Co3O4hybrid microelectrode to 1 and 10 μM glucose. (d) Glucose sensitivities of seamless S/NPG and fresh and reused S/NPG/Co3O4microelectrodes as a function of the concentration of glucose. Figure 4: Amperometric glucose detection. ( a ) Chronoamperometry curves and ( b ) the calibration curves (current density versus glucose concentration) for the amperometric responses of seamless S/NPG and fresh and reused S/NPG/Co 3 O 4 microelectrodes to the successive addition of glucose with the concentrations from 1 μM to 10 mM in 0.5 M KOH solution at a constant potential of 0.26 V (versus Ag/AgCl). ( c ) Fast response of seamless S/NPG/Co 3 O 4 hybrid microelectrode to 1 and 10 μM glucose. ( d ) Glucose sensitivities of seamless S/NPG and fresh and reused S/NPG/Co 3 O 4 microelectrodes as a function of the concentration of glucose. Full size image Figure 4 gives the typical comparisons of amperometric responses between bare S/NPG and S/NPG/Co 3 O 4 hybrid microelectrodes synthesized at the optimized alloying/dealloying and hydrothermal conditions (the first ones in Supplementary Table S1 ). Owing to the synergistic electrocatalytic activity of Au/Co 3 O 4 hybrid nanostructure and the excellent conductivity of seamless solid/nanoporous architecture, the amperometric response of the seamless S/NPG/Co 3 O 4 hybrid microelectrode exhibits perfect and stable step curve with dramatically enhanced current density in comparison with that of bare S/NPG ( Fig. 4a ). It should be noted that a response time no more than 1 s to research 95% of steady-state current ( Fig. 4c and Supplementary Fig. S16a ) is much faster than 2 s for nanometal-decorated graphite nanoplatelet [19] , 6 s for GOx-CNT networks [41] or 7 s for porous Co 3 O 4 nanofibers [15] . In consequence, incorporating Co 3 O 4 nanoparticles into the 3D bicontinuous nanoporous gold of seamless solid/nanoporous structure remarkably improves the glucose sensing ability compared with the bare seamless S/NPG microwire as well as free Co 3 O 4 nanoparticles ( Fig. 4a and Supplementary Fig. S13c ), which is further verified by their calibration curves ( Fig. 4b and Supplementary Fig. S13d ). As illustrated in the current density versus concentration plots ( Supplementary Figs S16–S18 ), the glucose biosensors based on Co 3 O 4 nanoparticles, seamless S/NPG and S/NPG/Co 3 O 4 hybrid microelectrodes show multi-linear detection ranges with different sensitivities up to 7, 30 and 70 mM, respectively, displaying a strong dependence on the concentration of added glucose ( Fig. 4d ). As the concentration decreases to 1 μM, the sensitivity of seamless S/NPG/Co 3 O 4 hybrid increases up to ~12.5 mA mM −1 cm −2 , much higher than the values of bare seamless S/NPG (0.72 mA mM −1 cm −2 ) ( Fig. 4d ) and Co 3 O 4 nanoparticles ( Supplementary Fig. S13 ). Such an ultrahigh sensitivity offers the seamless S/NPG/Co 3 O 4 microelectrode a remarkably low detection limit of 5 nM ( Fig. 5a ), much lower than some of the lowest values reported previously: 970 nM for electrospun Co 3 O 4 nanofibers [15] , 25 nM for 3D graphene/Co 3 O 4 composite [27] or 1.29 μM for the GOx-immobilized one-dimensional TiO 2 nanostructure [21] . Moreover, the seamless S/NPG/Co 3 O 4 microelectrode provides superb selectivity for glucose detection at the low applied potential of 0.26 V, which minimizes the responses of common interference species such as uric acid, acetamidophenol and ascorbic acid, in physiological levels [38] , [42] , as well as other sugars including fructose, mannose, maltose, sucrose and lactose [42] . Addition of 0.02 mM uric acid, 0.1 mM acetamidophenol, ascorbic acid or other sugars to a 1-mM glucose solution results in only ~0.5–5% increase in the current density, and does not interfere with the glucose detection even without the permselective coatings ( Fig. 5b and Supplementary Table S2 ). These predominant properties enlist this hybrid microelectrode to exhibit high reliability for analysing blood serums. 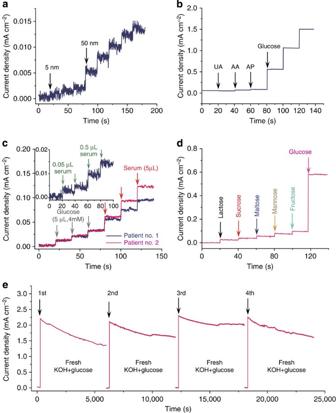Figure 5: Selectivity and stability. (a) Amperometric response to glucose with the low limit concentrations of 5 and 50 nM. Amperometric response to the successive addition of interfering compounds such as (b) 0.02 mM uric acid (UA), 0.1 mM acetamidophenol (AP), 0.1 mM ascorbic acid (AA) and (d) 0.1 mM fructose, mannose, maltose, sucrose, lactose, as well as 1 mM glucose at a potential of 0.26 V. (c) Current response of the S/NPG/Co3O4microelectrode to successive three-time additions of 5 μl glucose (4 mM) and blood serum of two diabetic patients into 20 ml 0.5 M electrolyte. Inset: Current response of the S/NPG/Co3O4microelectrode stored at room temperature for 4 months to ultralow concentration of serum. (e) Current-time curve for the S/NPG/Co3O4at 0.26 V in four fresh electrolytes containing 0.5 M KOH and 10 mM glucose. Figure 5c demonstrates the current-time curves for the successive additions of 5 μl 4 mM glucose standard solution and 5 μl blood serums of diabetic patients into 20 ml 0.5 M KOH solution, according to which the measured blood-glucose concentrations of diabetic patients are consistent with the values reported by the clinical analysis in the hospital ( Supplementary Table S3 ). Figure 5: Selectivity and stability. ( a ) Amperometric response to glucose with the low limit concentrations of 5 and 50 nM. Amperometric response to the successive addition of interfering compounds such as ( b ) 0.02 mM uric acid (UA), 0.1 mM acetamidophenol (AP), 0.1 mM ascorbic acid (AA) and ( d ) 0.1 mM fructose, mannose, maltose, sucrose, lactose, as well as 1 mM glucose at a potential of 0.26 V. ( c ) Current response of the S/NPG/Co 3 O 4 microelectrode to successive three-time additions of 5 μl glucose (4 mM) and blood serum of two diabetic patients into 20 ml 0.5 M electrolyte. Inset: Current response of the S/NPG/Co 3 O 4 microelectrode stored at room temperature for 4 months to ultralow concentration of serum. ( e ) Current-time curve for the S/NPG/Co 3 O 4 at 0.26 V in four fresh electrolytes containing 0.5 M KOH and 10 mM glucose. Full size image The electrochemical stability of the S/NPG/Co 3 O 4 hybrid microelectrode is investigated by the chronoamperometric method in four fresh solutions containing 0.5 M KOH and 10 mM glucose ( Fig. 5d ). In spite of the slow decrease of the current with time, the starting current response maintains stable in each fresh electrolyte, revealing the good stability of the hybrid microelectrodes during the electrochemical measurements. This is also confirmed by UV–visible spectrum of the measurement solution, where no Co or Au ion is detected ( Supplementary Fig. S19 ). Moreover, the aging tolerance ensures the S/NPG/Co 3 O 4 hybrid microelectrode to retain ~99.5% of its original current response over a storage period of 15 days at room temperature ( Supplementary Fig. S20 ), indicating the excellent reproducibility with a relative s.d. of ~0.6%. Even the S/NPG/Co 3 O 4 hybrid microelectrode stored at room temperature for 4 months still maintains the high capability to analyse serum sample at ultralow concentrations (inset of Fig. 5c ). To demonstrate the reusability, an S/NPG/Co 3 O 4 hybrid microelectrode is reconstructed via a procedure: etching the used S/NPG/Co 3 O 4 microelectrode in concentrated HNO 3 to remove Co 3 O 4 ( Supplementary Fig. S21a ), and then reincorporating Co 3 O 4 nanoparticles onto the used S/NPG microwire by hydrothermal method ( Supplementary Fig. S21b ). The amperometric response of the reused S/NPG/Co 3 O 4 microelectrode to the successive addition of glucose shows outstanding glucose sensing performance comparable to the as-prepared one ( Fig. 4a , and Supplementary Fig. S22 ), indicating its superior reusability and reproducibility. Thus, the seamless S/NPG/Co 3 O 4 hybrid microelectrode is an excellent material for the enhanced electrochemical sensing. In the perspective of the Langmuir isothermal theory for surface electrocatalytic reaction [15] , the sensitivity ( m ) of seamless S/NPG/Co 3 O 4 microelectrode is governed by the glucose concentration ( C g ) (as shown in Fig. 4d ), namely, m = di T / dC g = K B K A C a /(1+ K A C g ) [2] , where the total current density i T = K B C gS with C gS = K A C g C a /(1+ K A C g ) being the concentration of glucose adsorbed on the catalyst surface, C a denotes the molar concentration of active sites on the catalyst, K A and K B are the adsorption equilibrium constant and the reaction rate constant, respectively [15] . As C g is low enough (1 μM), that is, 1<< K A C g , m L ≈ K B K A C a =12.5 mA mM −1 cm −2 , indicating the intrinsically ultrahigh electrocatalytic activity of seamless S/NPG/Co 3 O 4 hybrid microelectrode towards glucose oxidation due to the unique nanoarchitecture of seamless S/NPG skeleton and synergistic Au/Co 3 O 4 hybrid. The seamless S/NPG framework, ingeniously integrating NPG layer with current collector by directly alloying/dealloying process on Au wire, minimizes the contact resistance between NPG layer and current collector, and thus optimizes the sensing performance in comparison with NPG species binded to current collector by polymer binders or adhesives ( Supplementary Fig. S23 ) [38] . Meanwhile, the 3D open and bicontinuous nanoporous structure provides a large room for loading Co 3 O 4 nanoparticles, and the produced nanoporous Au/Co 3 O 4 hybrid with extremely large specific surface area enhances the mass transport kinetics and facilitates sufficient use of the highly active Au/Co 3 O 4 hybrid [6] , [7] , [9] . Therefore, the thicker the NPG layer with the same characteristic length ( Supplementary Note 2 ), the higher the glucose sensitivity of S/NPG/Co 3 O 4 hybrid microelectrode ( Supplementary Fig. S24 ). Although free nanostructured Co 3 O 4 has intrinsically ultralow conductivity that limits its application in biosensing ( Supplementary Figs S13,S18 ) [15] , the nanoporous Au/Co 3 O 4 hybrid substantially enhances the electron transfer and improves the electrocatalytic activity of Co 3 O 4 ( m Co3O4 ), which is approximately calculated by subtracting the value of NPG ( m NPG ) according to the equation m Co3O4 = m L − m NPG =11.72 mA mM −1 cm −2 , two orders of magnitude higher than that of porous Co 3 O 4 nanofibers [15] . This great enhancement allows the seamless S/NPG/Co 3 O 4 microelectrode to detect glucose at ultralow concentrations with exquisite selectivity for potential applications in monitoring glucose in conventional and unconventional body fluids, as well as complementing or even replacing the GOx-based biosensors outside their rigorous operational environments (high temperature, high pH and so on). Additionally, the facile collection and reusability of S/NPG and S/NPG/Co 3 O 4 microwires can dramatically reduce the cost of Au/Co 3 O 4 -based biosensing devices, meeting low-cost requirements for the large-scale biosensing use. In summary, by the facile two-step procedure involving electrochemical alloying/dealloying and hydrothermal synthesis we have developed a seamless microelectrode with hybrid nanoarchitecture of S/NPG/Co 3 O 4 as a promising electrode material for high-performance electrochemical biosensors with ultrahigh sensitivity and ultrafast response time. The impressive glucose sensing behaviour of seamless S/NPG/Co 3 O 4 hybrid microelectrodes originates from the substantially enhanced electrocatalytic activity of the Au/Co 3 O 4 hybrid and the unique seamless solid/porous nanoarchitecture, which simultaneously minimizes the primary resistances in biosensing, viz. the electrochemical reaction occurring at electrode/electrolyte interfaces, the mass transport of analyte in electrolyte and electrode, and the electron conduction in electrode and current collector. Fabrication of seamless microwires The seamless S/NPG wires were prepared by a multicyclic electrochemical alloying/dealloying method based on a three-electrode electrochemical cell (Iviumstat electrochemical analyzer, Ivium Technology), in which Zn plate and wire were used as the auxiliary electrode and the reference electrode in a BA electrolyte containing 1.5 M ZnCl 2 , respectively [31] . 3D bicontinuous nanoporous layer with tunable microstructural features was decorated on polished Au wires with diameters of ~200 μm after the electrochemical cycles in the potential range from −0.72 to 1.88 V (versus Zn) at different conditions ( Supplementary Table S1 ) [31] . After acetone, ethanol and deionized water (18.2 MΩ cm) rinsing in sequence, the seamless S/NPG wire fixed on a plastic clamp was moved into the Teflon-lined stainless steel autoclave filled with the mixture of 3, 6, 9 mM Co(NO 3 ) 2 , 2 mM cetyltrimethylammonium bromide, 5 ml pure water and 30 ml ethanol. The sealed autoclave was heated in an electric oven at 100, 180 and 260 °C for 90 min for synthesis of the seamless Au/NPG/Co 3 O 4 ( Supplementary Table 1S ). After cooled to room temperature, the hybrid wire was washed with deionized water. The S/NPG microwire was collected from the tested S/NPG/Co 3 O 4 microelectrode via chemical etching in 60% HNO 3 for the further reconstruction of S/NPG/Co 3 O 4 microelectrode via hydrothermal method at the first conditions in Supplementary Table S1 . Characterization The microstructure and chemical composition of the specimens were investigated using a field-emission transmission electron microscope (JEOL JEM-2100F, 200 keV), and a field-emission scanning electron microscope (JEOL, JSM-6700F, 15 keV) equipped with an X-ray energy-dispersive microscopy. Raman spectrum was collected using a micro-Raman spectrometer (Renishaw) with a laser of 532 nm wavelength. X-ray diffraction measurement was carried out on a D/max2500pc diffractometer using Cu K α radiation. Electrochemical Measurement All cyclic voltammetry and amperometric experiments were performed in a three-electrode setup, which employed gold wire, seamless Au/NPG, Au/NPG/Co 3 O 4 microwires and Co 3 O 4 nanoparticles supported on ITO glass as the working electrodes, a Pt foil electrode as the counter electrode and a Ag/AgCl electrode as the reference electrode, in the 0.5 M KOH electrolyte bubbled by nitrogen gas for 30 min. The CVs were collected in the aqueous electrolyte with and without 10 mM glucose. The amperometric responses of microelectrodes to serum and glucose with different concentrations ranging from 1 μM to 10 mM were recorded under steady-state conditions at a potential of 0.26 V (versus Ag/AgCl). The concentration of blood glucose of diabetic patients was measured by automatic biochemical analyzer (Bakeman Coulter DXC800). How to cite this article: Lang, X.-Y. et al . Nanoporous gold supported cobalt oxide microelectrodes as high-performance electrochemical biosensors. Nat. Commun. 4:2169 doi: 10.1038/ncomms3169 (2013).